Two rotating cilia in the node cavity are sufficient to break left–right symmetry in the mouse embryo Determination of left–right asymmetry in mouse embryos is achieved by a leftward fluid flow (nodal flow) in the node cavity that is generated by clockwise rotational movement of 200–300 cilia in the node. The precise action of nodal flow and how much flow input is required for the robust read-out of left–right determination remains unknown. Here we show that a local leftward flow generated by as few as two rotating cilia is sufficient to break left–right symmetry. Quantitative analysis of fluid flow and ciliary rotation in the node of mouse embryos shows that left–right asymmetry is already established within a few hours after the onset of rotation by a subset of nodal cilia. Examination of various ciliary mutant mice shows that two rotating cilia are sufficient to initiate left–right asymmetric gene expression. Our results suggest the existence of a highly sensitive system in the node that is able to sense an extremely weak unidirectional flow, and may favour a model in which the flow is sensed as a mechanical force. The determination of left and right in the body plan is achieved by fluid flow in vertebrate embryos [1] with a few exceptions [2] . In the mouse embryo, breaking of left–right (L–R) symmetry is triggered at 7.75 days after fertilization (E7.75) by leftward flow in the node, an embryonic cavity at the midline that is filled with extraembryonic fluid [3] . The leftward fluid flow, referred to as nodal flow [4] , [5] , is generated by clockwise rotational movement of nodal cilia, each of which is a hair-like organelle that projects from the cell surface. The nodal cilia are tilted towards the posterior side and manifest both effective (leftward) and recovery (rightward) strokes, resulting in the net leftward flow [6] , [7] , [8] , [9] . Two principal hypotheses for the mechanism of flow action in L–R determination in the mouse embryo have been proposed. The two-cilia model suggests that two populations of nodal cilia exist in the node cavity: Motile cilia at the centre generate leftward flow, whereas immotile cilia in the perinodal region sense a mechanical signal from the flow [10] . The NVP model suggests that leftward flow transports submicrometer-sized vesicles (NVPs) that contain Sonic hedgehog and retinoic acid, which are essential for mouse embryogenesis [11] . Thus, although the role of nodal flow is well established in the mouse embryo, precisely how the flow functions in L–R determination remains unknown. Multiciliated cells constitute efficient mass transport systems in the airway, oviduct and subventricular zone of the brain in mice and humans [12] . Each multiciliated cell possesses hundreds of motile cilia that drive a global unidirectional fluid flow over long distances through planar beating. In contrast, each of the 200–300 ciliated cells in the node of mouse embryos has only a single motile cilium [8] . Although the node is a semi-closed structure that occupies a space much smaller than that of the airway or oviduct, it might be expected from the low density of cilia in the node that almost all of the node cilia would be necessary to generate a laminar unidirectional flow. We have now examined how the dynamics of nodal flow and L–R molecular patterning in the mouse embryo are affected when the number of cilia or the velocity of ciliary rotation is greatly reduced. Unexpectedly, we found that a weak flow generated by as few as two rotating cilia in the entire node cavity is sufficient for breaking of L–R symmetry. L–R asymmetry of Cerl2 is initiated when leftward flow is weak We first investigated the relationship between nodal flow and L–R determination in the mouse embryo. To study the dynamics of nodal flow, we measured its velocity distribution by particle image velocimetry (PIV) [8] , [13] ( Supplementary Movie 1 ). Time-lapse observations were performed during L–R axis determination with the use of a whole-embryo culture system [8] . At the early headfold (EHF) stage ( t =1 h), leftward fluid flow was locally generated in the node. At the two-somite stage ( t =10 h; Supplementary Movie 1 ), the directional flow was fully developed in the entire node. The nodal cilia continued to generate the net leftward flow during this time ( Fig. 1a ), with the net leftward velocity increasing about threefold to 3.0 μm s −1 between the EHF and two-somite stages ( Fig. 1b ). The cilia actually began to rotate and to generate the weak local flow at the EHF stage. Expression of Cerl2 in the perinodal region is bilateral at the EHF stage but becomes asymmetric (right-side dominant) at the late headfold (LHF) stage, soon after the local flow is generated and well before the global flow becomes maximal ( Fig. 1b,c ). These observations suggested that the flow begins to function at an early stage, possibly as early as the EHF stage, when the flow velocity is as low as 1.0 μm s −1 . They also suggest that Cerl2 is the earliest flow-responding gene, as previously described in the Xenopus embryo [14] . 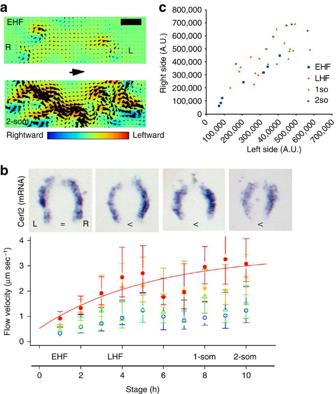Figure 1: AsymmetricCerl2expression is established when leftward flow is weak. (a) Velocity distribution of nodal flow in mouse embryos at the EHF and two-somite (2-som) stages. (b)Cerl2expression in the perinodal region (top panel) and leftward velocity of nodal flow (bottom panel) at various stages of development. The level of left-sided expression ofCerl2relative to that on the right is indicated by=(equal to) or < (less than). In the present study, we define 'local leftward flow' as the flow field with a leftward flow speed,U, in the range of 1.0–2.0 μm s−1. Red closed circles, blue open circles, orange asterisks, and green triangles denote velocity of L, R, posterior, and anterior directional flows, respectively. Values represent the 90th percentile (top 10th percentile) of the velocity distribution ±5% error bars. Three embryos were examined for analysis of flow velocity. (c) Quantification ofCerl2expression level in the node.Cerl2expression in the node was examined at various stages by whole mountin situhybridization. 1so, one somite stage; 2so, two-somite stage. The level ofCerl2expression on both sides of the node was quantified by measuring the pixel intensity of signals obtained by whole mountin situhybridization. Multiple embryos were examined for each stage;n=7 for EHF;n=12 for LHF;n=7 for one-somite;n=6 for two-somite. The L–R asymmetry inCerl2expression appears at the LHF stage (in∼50% of the LHF embryos). The black scale bar indicates 10 μm. The black arrow indicates 5 μm s−1. Figure 1: Asymmetric Cerl2 expression is established when leftward flow is weak. ( a ) Velocity distribution of nodal flow in mouse embryos at the EHF and two-somite (2-som) stages. ( b ) Cerl2 expression in the perinodal region (top panel) and leftward velocity of nodal flow (bottom panel) at various stages of development. The level of left-sided expression of Cerl2 relative to that on the right is indicated by=(equal to) or < (less than). In the present study, we define 'local leftward flow' as the flow field with a leftward flow speed, U , in the range of 1.0–2.0 μm s −1 . Red closed circles, blue open circles, orange asterisks, and green triangles denote velocity of L, R, posterior, and anterior directional flows, respectively. Values represent the 90th percentile (top 10th percentile) of the velocity distribution ±5% error bars. Three embryos were examined for analysis of flow velocity. ( c ) Quantification of Cerl2 expression level in the node. Cerl2 expression in the node was examined at various stages by whole mount in situ hybridization. 1so, one somite stage; 2so, two-somite stage. The level of Cerl2 expression on both sides of the node was quantified by measuring the pixel intensity of signals obtained by whole mount in situ hybridization. Multiple embryos were examined for each stage; n =7 for EHF; n =12 for LHF; n =7 for one-somite; n =6 for two-somite. The L–R asymmetry in Cerl2 expression appears at the LHF stage (in ∼ 50% of the LHF embryos). The black scale bar indicates 10 μm. The black arrow indicates 5 μm s −1 . Full size image Local weak leftward flow can establish L–R asymmetry To address directly whether the weak local flow functions in L–R determination, we prevented the leftward global flow with the use of a nontoxic viscous reagent (methylcellulose) as previously used for Xenopus embryos [15] . Whereas node cilia generated the leftward global flow in control medium, ciliary motion and fluid flow were abolished in medium containing 1.0% (w/v) methylcellulose. In the presence of an intermediate concentration (0.5%) of methylcellulose, the number of rotating cilia and the average rotating speed are significantly reduced, but the weak leftward local flow <2.0 μm s −1 was apparent ( Fig. 2a ; Supplementary Movie 2 ). To examine the effect of methylcellulose on L–R determination, we first cultured embryos at the EHF stage in the presence of 0, 0.5 or 1.0% methylcellulose for 5 h and then cultured them overnight in medium containing 1.0% methylcellulose to eliminate the effect of the later onset of leftward global flow. L–R asymmetric gene expression was monitored with the use of the Pitx2 ASE-lacZ transgene (which encodes β-galactosidase under the control of the left side–specific asymmetric enhancer of Pitx2 ) as a reporter [16] . In such experiments, ciliary motion, if it exists, would be limited to the first 5 h from the EHF stage. In the absence of flow throughout the culture period (treatment with 1.0% methylcellulose from the beginning), asymmetric gene expression was randomized ( Fig. 2b ). However, most of the embryos that were treated initially with 0.5% methylcellulose, in which the weak local flow was maintained, showed normal L–R asymmetric gene expression. When the incubation time for 5% methylcellulose was shortened to 2 h, asymmetric gene expression was still maintained ( Supplementary Fig. S1 ), suggesting that the presence the flow for 2 h is sufficient for symmetry breaking. These results suggested that the weak local flow is sufficient to initiate L–R asymmetric gene expression at the EHF stage. 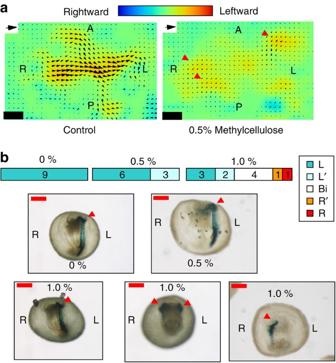Figure 2: Prevention of global leftward flow by methylcellulose. (a) Mouse embryos at the EHF stage were transferred to culture medium containing 0, 0.5 or 1.0% (w/v) methylcellulose, and the motility of node cilia and nodal flow were monitored. Whereas node cilia generated the leftward global flow in control medium (left panel), ciliary motion and fluid flow were completely lost in medium containing 1.0% methylcellulose. In the presence of 0.5% methylcellulose, the weak leftward local flow generated by ciliary rotation was observed (right panel). The black scale bars indicate 10 μm. Red arrowheads denote local leftward directional flow. A, anterior; P, posterior. (b) Mouse embryos harbouring thePitx2 ASE-lacZtransgene were isolated at the EHF stage, cultured in the presence of 0, 0.5, or 1.0% methylcellulose for 5 h, and then transferred to culture medium containing 1.0% methylcellulose and incubated for an extra 12 h. L–R asymmetric gene expression in the lateral plate was monitored with thePitx2 ASE-lacZtransgene as a reporter. L, L′, Bi, R′, and R denote exclusively left-sided, left side–dominant, bilateral, right side–dominant, and exclusively right-sided expression of the transgene, respectively. The numbers of embryos showing each phenotype are presented in the coloured boxes. Representative embryos stained with the β-galactosidase substrate X-gal are also shown, with the red arrowheads indicatinglacZexpression. The red scale bars indicate 1 mm. The black arrow indicates 5 μm s−1. Figure 2: Prevention of global leftward flow by methylcellulose. ( a ) Mouse embryos at the EHF stage were transferred to culture medium containing 0, 0.5 or 1.0% (w/v) methylcellulose, and the motility of node cilia and nodal flow were monitored. Whereas node cilia generated the leftward global flow in control medium (left panel), ciliary motion and fluid flow were completely lost in medium containing 1.0% methylcellulose. In the presence of 0.5% methylcellulose, the weak leftward local flow generated by ciliary rotation was observed (right panel). The black scale bars indicate 10 μm. Red arrowheads denote local leftward directional flow. A, anterior; P, posterior. ( b ) Mouse embryos harbouring the Pitx2 ASE-lacZ transgene were isolated at the EHF stage, cultured in the presence of 0, 0.5, or 1.0% methylcellulose for 5 h, and then transferred to culture medium containing 1.0% methylcellulose and incubated for an extra 12 h. L–R asymmetric gene expression in the lateral plate was monitored with the Pitx2 ASE-lacZ transgene as a reporter. L, L′, Bi, R′, and R denote exclusively left-sided, left side–dominant, bilateral, right side–dominant, and exclusively right-sided expression of the transgene, respectively. The numbers of embryos showing each phenotype are presented in the coloured boxes. Representative embryos stained with the β-galactosidase substrate X-gal are also shown, with the red arrowheads indicating lacZ expression. The red scale bars indicate 1 mm. The black arrow indicates 5 μm s −1 . Full size image Two motile cilia are sufficient for L–R symmetry breaking Screening of various ciliary mutants revealed an interesting phenotype for Dpcd and Rfx3 mutant embryos, which exhibit L–R patterning defects with an incomplete penetrance [17] , [18] . Pitx2 expression in the lateral plate is left-sided (7/13 embryos) or absent (6/13 embryos) in Dpcd −/− embryos, whereas it is left-sided (5/18 embryos), bilateral (8/18 embryos), right-sided (1/18 embryos) or absent (4/18 embryos) in Rfx3 −/− embryos ( Supplementary Fig. S2 ). We examined movement of node cilia and then the expression of L–R markers in individual embryos. Although the number of total node cells/cilia and was reduced only slightly (70–80% of the wild-type) in Dpcd and Rfx3 mutant embryos ( Fig. 3 ; Supplementary Fig. S3 ), their motility is greatly impaired ( Fig. 3 ). Most of the cilia in these mutants were either silent or showed slow planar beating instead of rotation, but a few rotating motile cilia remained ( Supplementary Movies 3 and 4 ; Fig. 3a–c and Supplementary Movies 5 , 6 , 7 ). The motility of node cilia were variably impaired in Dpcd and Rfx3 mutants: whereas four or five rotating motile cilia were observed in mildly affected embryos, only one or no motile cilia were apparent in severely affected embryos ( Fig. 4a–c,d–f ). In the severely affected embryos, expression of Cerl2 at the node was bilateral whereas left-sided Nodal expression in the lateral plate was lost ( Fig. 4b,e ; Supplementary Movies 8 and 9 ). Unexpectedly, however, L–R asymmetric expression of Cerl2 and Pitx2 was maintained in the mildly affected embryos, despite the fact that they have only four or five rotating cilia ( Fig. 4c,f ; Supplementary Movies 10 and 11 ). 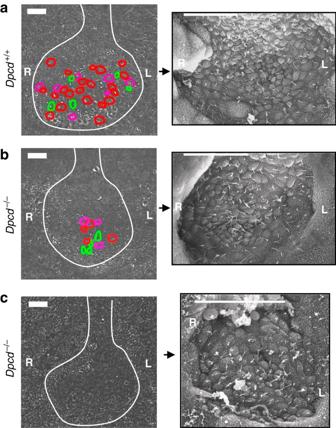Figure 3: Motility and morphology of nodal cilia inDpcdmutant embryos. (a–c) Motility and morphology of node cilia inDpcdmutant embryos. The wild type (a) (n=2) andDpcdmutant embryos (n=2) (b,c) were first subjected to ciliary motility assay (left panels) followed by scanning electron microscopy (right panels). Coloured circles indicate rotating cilia, with red and pink circles denoting posteriorly tilted cilia; green circles denote rotating cilia showing no tilt. The number of total rotating cilia in the node cavity was determined by changing the focal plane. Although all the rotating cilia are shown for the mutant embryos (b,c), only a portion of rotating cilia detected on a single plane is shown for the wild-type (+/+) embryos (a). The numbers of node cilia detected by scanning electron microscopy are 199 (a), 157 (b), and 141 (c), respectively. The white scale bars indicate 10 μm (left panels) and 20 μm (right panels), respectively. Figure 3: Motility and morphology of nodal cilia in Dpcd mutant embryos. ( a – c ) Motility and morphology of node cilia in Dpcd mutant embryos. The wild type ( a ) ( n =2) and Dpcd mutant embryos ( n =2) ( b , c ) were first subjected to ciliary motility assay (left panels) followed by scanning electron microscopy (right panels). Coloured circles indicate rotating cilia, with red and pink circles denoting posteriorly tilted cilia; green circles denote rotating cilia showing no tilt. The number of total rotating cilia in the node cavity was determined by changing the focal plane. Although all the rotating cilia are shown for the mutant embryos ( b , c ), only a portion of rotating cilia detected on a single plane is shown for the wild-type (+/+) embryos ( a ). The numbers of node cilia detected by scanning electron microscopy are 199 ( a ), 157 ( b ), and 141 ( c ), respectively. The white scale bars indicate 10 μm (left panels) and 20 μm (right panels), respectively. 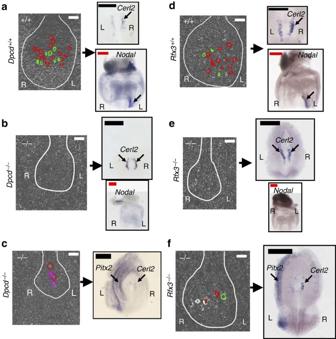Figure 4: Relation between dynamics of nodal cilia and L–R asymmetric gene expression inDpcdandRfx3mutant embryos. Ciliary motion and L–R marker gene expression were examined in the wild-type embryo (a), andDpcdmutant embryos with severe (b) or mild (c) impairment of the formation of motile node cilia. Similarly, the wild-type embryo (d), andRfx3mutant embryos with severe (e) or mild (f) impairment of the formation of motile node cilia were examined for ciliary motion and L–R marker gene expression. For each embryo, rotating cilia in the node are shown on the left, whereas expression pattern of L–R markers is shown in the right boxes. Rotating cilia are shown by coloured circles. Red and pink circles denote posteriorly tilted cilia, whereas green and white circles denote rotating cilia showing no tilt. The number of total rotating cilia in the node cavity was determined by changing the focal plane. Although all the rotating cilia are shown for the mutant embryos, only a portion of rotating cilia detected on a single plane is shown for the wild-type (+/+) embryos (a,d). Expression ofCerl2in the node and that ofNodalorPitx2in the lateral plate mesoderm were examined as L–R markers byin situhybridization. Asymmetric expression ofCerl2andPitx2was maintained in the mildly affected mutant embryos at the six-somite stage, whereas that ofCerl2andNodalwas lost in the severely affected embryos. The white, black and red scale bars indicate 10 μm, 70 μm and 0.5 mm, respectively. Full size image Figure 4: Relation between dynamics of nodal cilia and L–R asymmetric gene expression in Dpcd and Rfx3 mutant embryos. Ciliary motion and L–R marker gene expression were examined in the wild-type embryo ( a ), and Dpcd mutant embryos with severe ( b ) or mild ( c ) impairment of the formation of motile node cilia. Similarly, the wild-type embryo ( d ), and Rfx3 mutant embryos with severe ( e ) or mild ( f ) impairment of the formation of motile node cilia were examined for ciliary motion and L–R marker gene expression. For each embryo, rotating cilia in the node are shown on the left, whereas expression pattern of L–R markers is shown in the right boxes. Rotating cilia are shown by coloured circles. Red and pink circles denote posteriorly tilted cilia, whereas green and white circles denote rotating cilia showing no tilt. The number of total rotating cilia in the node cavity was determined by changing the focal plane. Although all the rotating cilia are shown for the mutant embryos, only a portion of rotating cilia detected on a single plane is shown for the wild-type (+/+) embryos ( a , d ). Expression of Cerl2 in the node and that of Nodal or Pitx2 in the lateral plate mesoderm were examined as L–R markers by in situ hybridization. Asymmetric expression of Cerl2 and Pitx2 was maintained in the mildly affected mutant embryos at the six-somite stage, whereas that of Cerl2 and Nodal was lost in the severely affected embryos. The white, black and red scale bars indicate 10 μm, 70 μm and 0.5 mm, respectively. Full size image To determine how much flow input the ciliary mutant embryos generate, we further investigated the relationship between the dynamics of nodal cilia, flow velocity distribution, and L–R marker gene expression in individual embryos at the four-to-six-somite stage ( Fig. 5 ). The severely affected embryos with no or one motile cilium showed no fluid flow as well as impaired L–R asymmetric gene expression ( Fig. 5a–f ). In contrast, embryos with two or more rotating cilia exhibited normal L–R patterning, with the exception of one embryo with five cilia ( Fig. 5g–v,w ). Those embryos with two-to-six rotating cilia lost global flow but showed the weak leftward flow ( Fig. 5h,k,n,q,t ), similar to wild-type embryos at the EHF stage ( Fig. 1a ). Although some cilia (for example, those in Fig. 5j,m ) in these embryos generated vortical flows, most rotating cilia generated leftward flow, suggesting that they are posteriorly tilted. Indeed, the posterior tilt of node cilia was maintained in the Rfx3 mutant embryos ( Supplementary Fig. S3 ). The weak flow that remained in the embryos with only two ( Fig. 5g ) or three ( Fig. 5j ) rotating cilia was 1.0 and 1.7 μm s −1 , respectively, in the area close to the cilia. However, the local flow decreased steeply with distance. The flow velocity at the edge of the node, where the flow-mediated signal is most likely received, was thus often too low to be detected by our method. 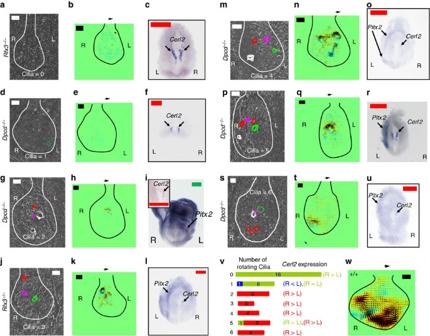Figure 5: Two rotating cilia are sufficient for L–R asymmetric gene expression inDpcdandRfx3mutant embryos. (a–u) The number of rotating cilia detected by a high-speed camera via transmitted light from a halogen lamp (a,d,g,j,m,p,s), flow velocity distribution (b,e,h,k,n,q,t), and L–R marker gene expression (c,f,i,l,o,r,u) were examined in individualDpcdandRfx3mutant embryos at the four-to-six-somite stages. The embryo shown in (a–c) is the same embryo shown inFigure 4e. Coloured circles indicate rotating cilia, with red and pink circles denoting posteriorly tilted cilia; green and white circles denote rotating cilia showing no tilt. Expression ofCerl2in the node and that ofPitx2in the lateral plate mesoderm were examined as L–R markers. Asymmetric expression ofCerl2andPitx2was maintained in the mildly affected mutant embryos (l,o,r,u). (v) Summary of the relation between the number of rotating cilia andCerl2expression. L–R asymmetricCerl2expression was impaired in embryos with no, or only one, rotating node cilium, whereas it was retained in those with two or more rotating cilia. (w) Flow velocity distribution for nodal flow in a wild-type (+/+) embryo at the four-somite stage. Global leftward flow is generated across the entire node cavity. The white and the black scale bars indicate 10 μm. The red and green scale bars indicate 70 μm and 0.5 mm, respectively. The black arrows indicate 5 μm s−1. Figure 5: Two rotating cilia are sufficient for L–R asymmetric gene expression in Dpcd and Rfx3 mutant embryos. ( a – u ) The number of rotating cilia detected by a high-speed camera via transmitted light from a halogen lamp ( a , d , g , j , m , p , s ), flow velocity distribution ( b , e , h , k , n , q , t ), and L–R marker gene expression ( c , f , i , l , o , r , u ) were examined in individual Dpcd and Rfx3 mutant embryos at the four-to-six-somite stages. The embryo shown in ( a – c ) is the same embryo shown in Figure 4e . Coloured circles indicate rotating cilia, with red and pink circles denoting posteriorly tilted cilia; green and white circles denote rotating cilia showing no tilt. Expression of Cerl2 in the node and that of Pitx2 in the lateral plate mesoderm were examined as L–R markers. Asymmetric expression of Cerl2 and Pitx2 was maintained in the mildly affected mutant embryos ( l , o , r , u ). ( v ) Summary of the relation between the number of rotating cilia and Cerl2 expression. L–R asymmetric Cerl2 expression was impaired in embryos with no, or only one, rotating node cilium, whereas it was retained in those with two or more rotating cilia. ( w ) Flow velocity distribution for nodal flow in a wild-type (+/+) embryo at the four-somite stage. Global leftward flow is generated across the entire node cavity. The white and the black scale bars indicate 10 μm. The red and green scale bars indicate 70 μm and 0.5 mm, respectively. The black arrows indicate 5 μm s −1 . Full size image We also examined the effects of methylcellulose on the L–R patterning of Dpcd mutant embryos ( Fig. 6 ). Treatment of wild-type embryos with 0.5% methylcellulose for 12 h, which greatly reduces the number of rotating cilia ( Fig. 6a ) and the rotation speed, still maintained correct L–R patterning, as revealed by L–R asymmetric distribution of phosphorylated Smad2/3 in the lateral plate ( n =7, Fig. 6c ). When Dpcd −/− embryos that possessed <>3 rotating cilia in the absence of methylcellulose were similarly treated with 0.5% methylcellulose, however, the L–R asymmetry in the level of phosphorylated Smad2/3 was lost ( n =2, Fig. 6d ), suggesting that the L–R decision depends on the flow generated by rotating cilia. 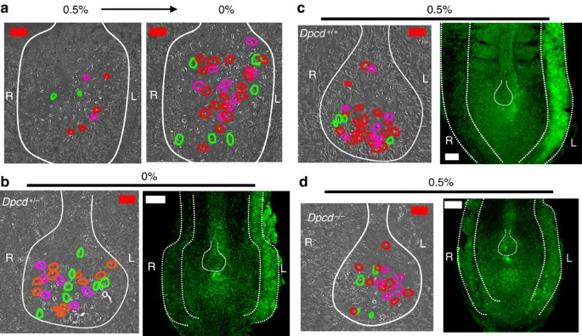Figure 6: Effects of methylcellulose on the L–R decision inDpcdmutant embryos. (a) Number of rotating cilia was examined in the presence of 0.5% methylcellulose, and after methylcellulose was removed. Coloured circles in left panels indicate rotating cilia, with red and pink circles denoting posteriorly tilted cilia; green circle denote rotating cilia showing no tilt. (b–d) Embryos with the indicated genotype were incubated without (b) or with 0.5% methylcellulose (c,d) for 12 h. They were first examined for the motility of nodal cilia in a short time (5–10 min), then were fixed with 4% paraformaldehyde for immunostaining with an antitibody specific to phosphorylated Smad2/3. Rotating cilia are shown in left panels, while distribution of phosphorylated Smad2/3 is shown in right panels. The colour codes of rotating cilia are the same as those in (a). Although all the rotating cilia are shown for theDpcd−/−embryos (d), only a portion of rotating cilia detected on a single plane is shown for theDpcd+/+(c) andDpcd+/−(b) embryos. The dotted lines in right panels denote the position of the lateral plate and the node. The L–R asymmetric distribution of phosphorylated Smad2/3 was maintained in (b) and (c) but was lost in (d). The red and the white scale bars indicate 10 and 50 μm, respectively. Figure 6: Effects of methylcellulose on the L–R decision in Dpcd mutant embryos. ( a ) Number of rotating cilia was examined in the presence of 0.5% methylcellulose, and after methylcellulose was removed. Coloured circles in left panels indicate rotating cilia, with red and pink circles denoting posteriorly tilted cilia; green circle denote rotating cilia showing no tilt. ( b – d ) Embryos with the indicated genotype were incubated without ( b ) or with 0.5% methylcellulose ( c , d ) for 12 h. They were first examined for the motility of nodal cilia in a short time (5–10 min), then were fixed with 4% paraformaldehyde for immunostaining with an antitibody specific to phosphorylated Smad2/3. Rotating cilia are shown in left panels, while distribution of phosphorylated Smad2/3 is shown in right panels. The colour codes of rotating cilia are the same as those in ( a ). Although all the rotating cilia are shown for the Dpcd −/− embryos ( d ), only a portion of rotating cilia detected on a single plane is shown for the Dpcd +/+ ( c ) and Dpcd +/− ( b ) embryos. The dotted lines in right panels denote the position of the lateral plate and the node. The L–R asymmetric distribution of phosphorylated Smad2/3 was maintained in ( b ) and ( c ) but was lost in ( d ). The red and the white scale bars indicate 10 and 50 μm, respectively. Full size image Finally, we examined the relationship between the position of node cilia and L–R gene expression in Dpcd mutant embryos ( Fig. 7a,n ). Those embryos with two or three rotating cilia exhibited normal L–R gene expression irrespective of the positions of the cilia with regard to the node cavity. Thus, normal L–R asymmetric expression of Cerl2 and Pitx2 was maintained whether the two or three motile cilia were located at the centre ( Fig. 7i,j ) or on the right side ( Fig. 7k,l ) of the node cavity. In embryos with only one motile cilium, on the other hand, L–R asymmetric gene expression was always lost regardless of the position of the cilium ( Fig. 7a–h ). Immotile cilia in the perinodal region, which have been proposed to sense nodal flow, were detected in the embryos with two or more rotating cilia, but they were present at a greatly reduced number compared with wild-type embryos ( Fig. 7i,k,m ). It was not possible to determine the precise number of immotile cilia, because they are difficult to detect with the microscopy system used. However, our results suggest that several immotile cilia are sufficient for sensing the flow-mediated signal. In this case, a mechanism that propagates the signal received by a few cells to all perinodal cells must exist. Overall, our results suggest that the weak leftward flow generated by as few as two motile cilia is sufficient to initiate asymmetric gene expression at the EHF stage and to establish L–R asymmetry in the mouse embryo. Inv mutant mouse exhibits slow leftward flow [19] and shows reversal of laterality [20] . L–R defects of Inv mutant may involve impaired flow and extra features [21] . 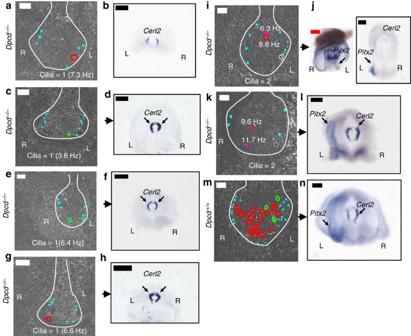Figure 7: L–R patterning is determined by the number of motile cilia inDpcdmutant embryos. (a–h) Relation between the position of one motile cilium and L–R asymmetric gene expression inDpcdmutant embryos at the four-to-six-somite stages. (i–l) Relation between the position of two motile cilia and L–R asymmetric gene expression inDpcdmutant embryos at the nine and the six-somite stages. (m,n) Relation between the position of motile cilia and L–R asymmetric gene expression in a wild-type (+/+) embryo at the six-somite stage. Coloured circles indicate rotating cilia, with red and pink circles denoting posteriorly tilted cilia; green and white circles denote rotating cilia showing no tilt. Although all the rotating cilia are shown for the mutant embryos (a,c,e,g,i,k), only a portion of rotating cilia detected on a single plane is shown for the wild-type (+/+) embryos (m). Cyan dots denote immotile cilia in the perinodal region. The white, black and red scale size bars indicate 10 μm, 50 μm and 0.5 mm, respectively. Figure 7: L–R patterning is determined by the number of motile cilia in Dpcd mutant embryos. ( a – h ) Relation between the position of one motile cilium and L–R asymmetric gene expression in Dpcd mutant embryos at the four-to-six-somite stages. ( i – l ) Relation between the position of two motile cilia and L–R asymmetric gene expression in Dpcd mutant embryos at the nine and the six-somite stages. ( m , n ) Relation between the position of motile cilia and L–R asymmetric gene expression in a wild-type (+/+) embryo at the six-somite stage. Coloured circles indicate rotating cilia, with red and pink circles denoting posteriorly tilted cilia; green and white circles denote rotating cilia showing no tilt. Although all the rotating cilia are shown for the mutant embryos ( a , c , e , g , i , k ), only a portion of rotating cilia detected on a single plane is shown for the wild-type (+/+) embryos ( m ). Cyan dots denote immotile cilia in the perinodal region. The white, black and red scale size bars indicate 10 μm, 50 μm and 0.5 mm, respectively. Full size image Flow-mediated signals, whether they are mechanical or chemical, are likely sensed by perinodal cells, which are ciliated cells located at the edge of the node. Indeed, we detected immotile cilia in the perinodal region of Dpcd and Rfx3 mutant embryos that possess only two motile cilia in the present study. In Xenopus , leftward flow is essential on the left side but dispensable on the right side of the gastrocoel roof plate for breaking L–R symmetry [22] , suggesting that the flow is sensed by cells on the left side of the roof plate. Similarly, it may be the cells on the left side of the node that sense the flow in mouse embryos. In the Dpcd and Rfx3 mutant embryos with two or three rotating cilia, we were able to detect the locally generated weak flow but were unable to observe it reaching the edge of the node. In some embryos ( Fig. 5j–l,p–r ), normal L–R patterning was maintained despite the fact that local flow was detected exclusively on the right half of the node cavity. However, the travelling flow in such embryos was likely too slow to be detected by our method. We expect that the weak leftward flow that occurred at the right side of the node was transmitted to the left side, given that the node cavity of the mouse embryo is covered by Reichert's membrane [23] , which renders the cavity a semi-closed space. Whether the action of nodal flow is to generate mechanical stress or to transport an unknown determinant molecule is a long-standing question. Our unexpected observation that a weak flow generated by as few as two rotating cilia is sufficient to break L–R symmetry does not rigorously distinguish between these two models, but it favours the mechanical force model. In terms of hydrodynamics on the microscopic scale, the slow leftward flow would still be expected to be capable of transporting molecules or particles across the node cavity. However, the flow generated by two rotating cilia is highly local ( Fig. 5h ), and under conditions with a low Reynolds number, when viscosity dominates and inertia is negligible, the flow velocity would be attenuated over a distance from the rotating cilia by a factor of 2–3. It would therefore take a relatively long time for a molecule or particle to travel from one side of the node to the other side. Alternatively, a weak mechanical force generated by such a slow flow may be sufficient to be sensed by the cells at the edge of the node. Theoretically, mechanical force can be transmitted essentially instantly (at the speed of sound) from the rotating cilia to the edge of the node, because the node cavity is a semi-closed space [24] . Such a scenario would explain our observation that a few rotating cilia can break L–R symmetry regardless of their positions. Primary cilia are able to behave as highly sensitive mechanical sensors [25] , [26] . As previously suggested in the two-cilia model [10] , [27] , we found that most of the primary cilia of the perinodal cells are immotile (S.Y., unpublished observations). We detected immotile cilia in the perinodal region of Dpcd or Rfx3 mutant embryos with only two or three rotating cilia, although their numbers were greatly reduced. For immotile cilia at the edge of the node to act as mechanical sensors, a mechanism that expands a signal received by a few individual cells to all perinodal cells would be required. Whether nodal flow is sensed as a mechanical force, or it transports a chemical determinant, our results suggest that the mouse node possesses a highly sensitive system that is able to detect an extremely weak signal generated by a slow flow. Animals Animals were maintained in the Animal Facility of Graduate School of Frontier Biosciences, Osaka University at 12:12 light cycle and were provided with food and water ad libitum . All experiments were approved by the Institutional Animal Care and Use Committee of the Osaka University.Wild-type embryos of timed pregnant ICR mice (CLEA Japan) were used for time-lapse observations. C57B6J ( Dpcd , Rfx3 ) and C57B6J/129 ( Dpcd ) mice were studied as ciliary mutants. Embryo dissection and whole-embryo culture Mouse embryos were dissected into phenol red-free DMEM supplemented with 10% fetal bovine serum (Invitrogen). The developmental stage (from EHF to two-somite) of embryos was determined on the basis of morphology and the number of somites. Dissected embryos were cultured at 37 °C in phenol red-free DMEM supplemented with 75% rat serum (Invitrogen). Observation of nodal flow and PIV analysis To characterize the flow fields of nodal flow, we used multipoint scanning confocal microscopy and PIV analysis. The node cavity was filled with phenol red-free DMEM supplemented with 10% fetal bovine serum and fluorescent microbeads (diameter of 0.2 μm, with excitation and emission wavelengths of 505 and 515 nm; Invitrogen). Motion of the beads was observed for 10 s (30 frames per second) at planes positioned 5, 10, 15 or 20 μm below the apical cell surface of the node cavity with the use of a CSU-X confocal unit (Yokogawa) and an iXon EMCCD camera (Andor Technology) connected to a DMI6000B microscope (Leica) with a ×60 glycerin-immersion objective lens. Time-series images for PIV analysis were captured at a resolution of 512 by 512 pixels and were processed with interrogation windows of 16 by16 pixels with 50% overlap, corresponding to a spatial resolution of 4.3 by 4.3 μm. To calculate the vector fields, we applied an iterative cross-correlation method. The time-averaged velocity distributions were calculated over 10 s. In our method, the lower limit of detectable velocity was 0.8 μm s −1 . High-speed imaging of nodal ciliary rotation To characterize the dynamic properties of nodal ciliary rotation, we used a high-speed camera and a point-tracking system. The node cavity was filled with phenol red-free DMEM supplemented with 10% fetal bovine serum, and rotation of the node cilia was observed at the apical cell surface of the node cavity for 2 s (100 frames s −1 ) with the use of a high-speed CMOS camera (HAS-500M, Detect). The camera was connected to an Axiovert 2 microscope for observation of individual node sections, the microscope being equipped with a ×100 oil-immersion objective lens. The specimen was observed with transmitted light from a halogen lamp. Time-series images were captured at a resolution of 1,024 by 992 pixels, with a pixel resolution of 0.082 by 0.082 μm. To visualize the outline of nodal cilia, we first subtracted the average image from the time-series images and enhanced contrast with 0.5% saturated pixels (ImageJ, NIH). We then detected the edges of nodal cilia by manual tracking with the use of image processing software (TEMA, Photron). As rotating cilia are located on multiple focal planes of the node cavity, the number of rotating cilia in the node was determined by examining various focal planes. Analysis of directional flow and its curve fitting Leftward ( V l ), rightward ( V r ), upward ( V a ), and downward ( V p ) directional flows for each developmental stage were calculated in the area that includes all directional flows and vortices. The velocities V l , V r , V a and V p were defined from the 90th and 10th percentile values of the velocity vector components in the positive or negative directions of the x axis and y axis, respectively. Analysis of ciliary rotation and asymmetric gene expression To examine the relationship among the dynamics of nodal cilia, flow velocity distribution, and L–R asymmetric gene expression, we measured all three parameters in the same individual embryos. Embryos were first examined for ciliary movement and fluid flow in a short time (5–15 min), and were subsequently fixed with 4% paraformaldehyde for in situ hybridization. For live imaging, the distal portions including the node cavity was dissected out from E8.0 mouse embryos. The level of phosphorylated Smad2/3 was examined with an antibody, specific to phosphorylated Smad2/3 (ref. 28 ): Mouse embryos were recovered and fixed for 2–12 h at 4 °C with 4% paraformaldehyde in PBS. They were then dehydrated with methanol and incubated for 1 h at room temperature with 3% H 2 O 2 in methanol. After rehydration with PBS containing 0.1% Triton X–100, they were incubated with blocking buffer (BB: 0.5% TSA Blocking Reagent (Perkin Elmer), 0.1 M Tris–HCl (pH7.5), 0.15MnaCl) before exposure to rabbit polyclonal antibodies to phosphorylated Smad2/3 (pSmad2) that can detect Smad3 phosphorylated at Ser465 and Ser467, and may detect phosphorylated Smad3 at its equivalent site (Cell Signaling Technology, #3101) at dilutions of 1:50 in BB. Immune complexes for pSmad2 were detected with biotinylated goat antibodies to rabbit immunoglobulinG (Vector) at a dilution of 1:200 in BB, a Vectastain ABC Kit (Vector), and fluorophore tyramide working solution (Perkin Elmer). In the wild-type embryo, distribution of phosphorylated Smad2/3 is L>>R in the node and L + R − in the lateral plate [28] . Quantification of Cerl2 expression in the node cells To quatify the levels of Cerl2 expression in the node cells, the pixel intensity of the signal obtained by whole mount in situ hybridization was measured. How to cite this article: Shinohara K. et al . Two rotating cilia in the node cavity are sufficient to break left–right symmetry in the mouse embryo. Nat. Commun. 3:622 doi: 10.1038/ncomms1624 (2012).